Morphological and functional remodelling of the neuromuscular junction by skeletal muscle PGC-1α The neuromuscular junction (NMJ) exhibits high morphological and functional plasticity. In the mature muscle, the relative levels of physical activity are the major determinants of NMJ function. Classically, motor neuron-mediated activation patterns of skeletal muscle have been thought of as the major drivers of NMJ plasticity and the ensuing fibre-type determination in muscle. Here we use muscle-specific transgenic animals for the peroxisome proliferator-activated receptor γ co-activator 1α (PGC-1α) as a genetic model for trained mice to elucidate the contribution of skeletal muscle to activity-induced adaptation of the NMJ. We find that muscle-specific expression of PGC-1α promotes a remodelling of the NMJ, even in the absence of increased physical activity. Importantly, these plastic changes are not restricted to post-synaptic structures, but extended to modulation of presynaptic cell morphology and function. Therefore, our data indicate that skeletal muscle significantly contributes to the adaptation of the NMJ subsequent to physical activity. The neuromuscular junction (NMJ) is a complex structure that mediates the cross-talk between motor neurons and muscle fibres. The embryonic and post-natal installation of NMJs has been studied extensively and the key factors that regulate the NMJ assembly in this context have been described, including agrin and acetylcholine, membrane protein complexes and extracellular matrix components as well as various neurotrophic factors [1] , [2] , [3] . At least some of these regulators are also responsible for guiding NMJ formation in denervation–reinnervation cycles that are observed in fibre damage, several muscle dystrophies or in the aging process [4] , [5] . Interestingly, while a dominant role for motor neurons in NMJ formation has been postulated, an increasing amount of evidence highlights the important contribution of skeletal muscle to the proper installation of the NMJ [2] , [6] , [7] , [8] . For example, prepatterning by primitive, aneural acetylcholine receptor (AChR) clusters on the muscle fibre membrane might help axonal guidance [9] . Likewise, skeletal muscle-specific receptor tyrosine-protein kinase (MuSK) and low-density lipoprotein receptor-related protein 4, two key components involved in post-synaptic agrin action, mediate retrograde signaling from the muscle to the motor neuron that is crucial for presynaptic differentiation of the NMJ during embryonic and postnatal development [10] . At least studies in Drosophila suggest that these proteins might also be involved in late-stage NMJ plasticity [11] ; however, this hypothesis remains to be substantiated in Drosophila as well as in vertebrates. Curiously, in contrast to the widely accepted important contribution of the skeletal muscle to NMJ formation in development and re-innervation, the role of this organ in mediating plastic changes of the mature NMJ is much less appreciated. For example, morphological and functional adaptations of the NMJ to endurance training improve neuromuscular transmission and thereby contribute to an increased fatigue resistance [12] , [13] . The neuromuscular exercise plasticity however has almost exclusively attributed to the rate and amplitude of myocellular calcium transients that are triggered by distinct patterns of motor neuron firing [14] , [15] . Thus, exercise adaptations of the NMJ that ultimately lead to a metabolic and myofibrillar fibre-type switch towards oxidative, high endurance muscle fibres are thought to be dominantly controlled by the neuronal input [16] . Accordingly, the plastic changes of NMJs in the trained neuromuscular context have been extensively characterized and include adaptations in endplate size, sprouting of nerve terminal branches, and electrophysiological kinetics [17] , [18] , [19] . However, the anterograde and retrograde signals involved in this remodelling remain largely enigmatic. Similarly, potential contributions of the skeletal muscle to these plastic changes have not been studied. Overexpression of the peroxisome proliferator-activated receptor γ co-activator 1α (PGC-1α) in cultured muscle cells is sufficient to promote postsynaptic NMJ gene transcription and the formation of aneural AChR clusters. Moreover, skeletal muscle-specific gain- and loss-of-function mouse models for PGC-1α exhibit altered expression of postsynaptic NMJ genes in muscle in vivo [20] . However, the consequence of altered muscle PGC-1α expression on NMJ morphology and function in vivo has not been assessed to date. Besides controlling postsynaptic NMJ gene expression, PGC-1α is a key regulatory nexus of endurance exercise adaptation in the skeletal muscle. Accordingly, PGC-1α levels are strongly regulated by physical activity [21] . Upon activation, PGC-1α promotes many, if not all of the adaptations of muscle to endurance training, including increased mitochondrial biogenesis and oxidative metabolism, vascularization and a switch towards type I and IIa oxidative, high-endurance muscle fibres [22] , [23] , [24] . Inversely, muscle-specific PGC-1α knockout mice exhibit features of pathological inactivity such as a switch towards glycolytic muscle fibres, reduced exercise capacity, fibre damage and local as well as systemic inflammation [25] , [26] . On the basis of the ability to promote a trained phenotype even in inactive muscle, overexpression of PGC-1α exerts a beneficial therapeutic effect in different contexts of muscular wasting, including Duchenne muscular dystrophy [20] , denervation-induced fibre atrophy, statin-mediated muscle dysmorphology, sarcopenia [27] or amyotrophic lateral sclerosis [28] , [29] . To assess the contribution of skeletal muscle to the plasticity of adult NMJ morphology and function, we now studied the muscle-specific PGC-1α transgenic mice as a genetic model for endurance exercise. Even though these animals exhibit a trained phenotype, the PGC-1α transgenics are not hyperactive and hence do not exhibit increased motor neuron firing when kept in a sedentary state [30] . This allows a dissociation of the effects from skeletal muscle and motor neurons on the NMJ in a mouse model of endurance exercise. Surprisingly, our findings demonstrate a hitherto underappreciated role for skeletal muscle to modulate NMJ plasticity both post- and pre-synaptically by improving NMJ integrity and function. Thus, in the adult neuromuscular system, shifts in the phenotype of the muscle fibres significantly contribute to the NMJ remodelling by activating a novel retrograde signalling. Transgenic PGC-1α expression in different tissues In the transgenic animals, the expression of PGC-1α is driven by the muscle creatine kinase (MCK) promoter. To ensure muscle specificity of expression, we measured PGC-1α expression in the MCK mice using the WT samples as reference. As expected, the relative PGC-1α mRNA expression was highest in the predominantly glycolytic muscles tibialis anterior (TA), extensor digitorum longus (EDL), sternocleidomastoid (SCM) and levator auris longus (LAL), followed by the more mixed muscle beds in gastrocnemius and diaphragm ( Fig. 1 ). The overexpression of PGC-1α was not significantly elevated in MCK mice in the oxidative soleus and transversus abdominis (TVA) muscles. Important for the present study, neuronal tissue, including spinal cord and brain, exhibited indistinguishable levels of PGC-1α transcript in WT and MCK animals, thus confirming the muscle specificity of the transgenic PGC-1α expression in this mouse line. 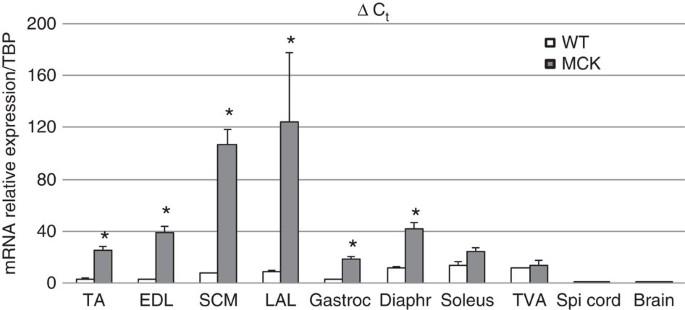Figure 1: Level of expression of PGC-1α in different muscles from WT and MCK mice Relative PGC-1α mRNA levels in tissues from WT (white bars,n=3) and MCK-PGC-1α mice (grey bars,n=3) (6- to 8-week-old). Total RNA was reverse transcribed and the level of expression of PGC-1α was determined by real-time PCR, relative to the TATA-Binding Protein (TBP) expression level, analysed according to the ΔCtmethod. Each bar represents mean±s.e.m. *P<0.05 (n=3,t-test two-tailed). TA: tibialis anterior, EDL: extensor digitorum longus, SCM: sternocleidomastoidian, LAL: levator auris longus, Gastroc: gastrocnemius, Diaphr: diaphragm, TVA: transversus abdominis. Figure 1: Level of expression of PGC-1α in different muscles from WT and MCK mice Relative PGC-1α mRNA levels in tissues from WT (white bars, n =3) and MCK-PGC-1α mice (grey bars, n =3) (6- to 8-week-old). Total RNA was reverse transcribed and the level of expression of PGC-1α was determined by real-time PCR, relative to the TATA-Binding Protein (TBP) expression level, analysed according to the Δ C t method. Each bar represents mean±s.e.m. * P <0.05 ( n =3, t- test two-tailed). TA: tibialis anterior, EDL: extensor digitorum longus, SCM: sternocleidomastoidian, LAL: levator auris longus, Gastroc: gastrocnemius, Diaphr: diaphragm, TVA: transversus abdominis. Full size image Elevated muscle PGC-1α modifies NMJ morphology The effect of muscle PGC-1α on postsynaptic gene expression in muscle cells and on formation of aneural AChR clusters in vitro has been demonstrated previously [20] . We now studied the consequences of elevated expression of PGC-1α in skeletal muscle on NMJ morphology in vivo . AChR aggregates in the post-synaptic membrane, typically pretzel-shaped, were stained with AF488-α-bungarotoxin (α-Bgtx), a very potent ligand for AChR (visualized in green). The motor neuron was labelled using an anti-neurofilament antibody revealed by a cyanin 5-conjugated secondary antibody (shown in red; Fig. 2a ). Quantification of the AChR clusters revealed a significantly smaller area in the glycolytic EDL and SCM of the MCK mice compared with their WT littermates ( Fig. 2b ). In contrast, the already smaller area of the postsynaptic endplates in the more oxidative diaphragm and soleus muscles was unchanged between MCK and WT animals ( Fig. 2b ). 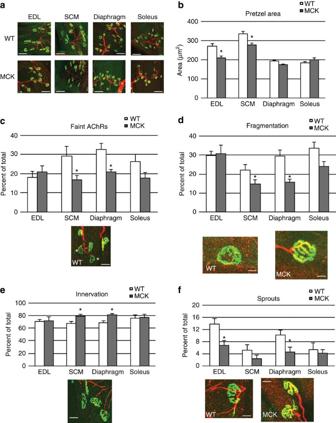Figure 2: Structural comparison of the NMJ from WT and transgenic mice. (a) Representative confocal stack image of fluorescently labelled NMJ in different muscles. Muscles were stained with AF488-coupled α-bungarotoxin to visualize AChRs (green) and anti-neurofilament antibodies coupled to cyanin 5 to stain the nerve part (red). Calibration bar: 200 μm (b) Mean area of the AChRs aggregates was determined using the Image J in arbitrary units. Each bar represents mean±s.e.m. *P<0.05 (N=3,t-test two-tailed). (c–f) The frequency of faint AChRs clusters, highlighted by a white star Calibration bar: 50 μm (c), fragmented AChRs clusters Calibration bar: 1.5 μm (d), innervated pretzels Calibration bar: 40 μm (e) and sprouted AChRs clusters Calibration bar: 25 μm (f) was determined on confocal images stack. Each bar represents mean±s.e.m. from at least 100 NMJ from three mice *P<0.05 (N=3,n>100,t-test two-tailed). White bars represent s animals, grey bars represent transgenic mice. Figure 2: Structural comparison of the NMJ from WT and transgenic mice. ( a ) Representative confocal stack image of fluorescently labelled NMJ in different muscles. Muscles were stained with AF488-coupled α-bungarotoxin to visualize AChRs (green) and anti-neurofilament antibodies coupled to cyanin 5 to stain the nerve part (red). Calibration bar: 200 μm ( b ) Mean area of the AChRs aggregates was determined using the Image J in arbitrary units. Each bar represents mean±s.e.m. * P <0.05 ( N =3, t- test two-tailed). ( c–f ) The frequency of faint AChRs clusters, highlighted by a white star Calibration bar: 50 μm ( c ), fragmented AChRs clusters Calibration bar: 1.5 μm ( d ), innervated pretzels Calibration bar: 40 μm ( e ) and sprouted AChRs clusters Calibration bar: 25 μm ( f ) was determined on confocal images stack. Each bar represents mean±s.e.m. from at least 100 NMJ from three mice * P <0.05 ( N =3, n >100, t- test two-tailed). White bars represent s animals, grey bars represent transgenic mice. Full size image NMJs always present a certain percentage of abnormalities at the post- and pre-synaptic levels. For example, the pretzel shape can be irregular, fragmented or the density of the clusters can be faint, a sign of decreased AChR intensity. The percentage of structural NMJ deformities increases as the mouse ages and can be rectified by caloric restriction or exercise [18] . Similar to the improvement mediated by these interventions, the post-synaptic architecture of the NMJs was also significantly improved in the young MCK mice ( Fig 2c–f ). In particular, SCM and diaphragm muscles of MCK animals displayed a reduction of faint pretzels ( Fig. 2c ) and the number of fragmented clusters ( Fig. 2d ) when compared with the WT counterparts, while no significant differences were detectable in EDL and soleus muscles. Likewise, overexpression of PGC-1α in skeletal muscle increased the number of innervated NMJs with clear co-localization of the AChR and the motor neuron signal in SCM and diaphragm ( Fig. 2e ) as well a reduction of sprouts, nerve terminals that do not terminate within an AChR cluster in EDL and diaphragm ( Fig. 2f ) of MCK mice. PGC-1α-mediated changes in the ultrastructure of the NMJ Our data indicate that muscle PGC-1α improves NMJ morphology on the histological level. Importantly, structural and functional stabilization of the NMJ is to a large extent governed by the total area of interface between the motor neuron and the muscle and hence the number and size of synaptic folds. 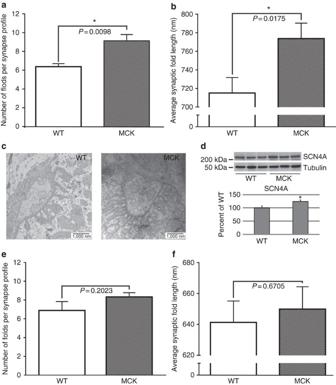Figure 3: Synaptic fold characterization on the TEM images from WT and transgenic mice NMJs. (a) The average number of folds attached to synapses was determined for WT and MCK mice in SCM muscle. (b) Synaptic fold lengths from SCM muscles were scaled and measured with Image J and averaged. Each bar represents mean±s.e.m. (n=4,t-test two-tailed). (c) Representative TEM image of the NMJ area of SCM muscle from WT or MCK animals. (d) Western blot detection of the Nav1.4 expression in SCM muscles from WT and MCK animals. The relative band intensity was analysed using the Image J. The WT/tubulin ratio was set as 100%. (e) The average number of folds attached to synapses was determined for WT and MCK mice in soleus muscle. (f) Synaptic fold lengths from soleus muscles were scaled and measured with Image J and averaged. Each bar represents mean±s.e.m. (n=4,t-test two-tailed). SF: Synaptic folds, m: mitochondria. Therefore, to investigate how PGC-1α expression in muscle could affect NMJ structure, we studied the synaptic folds on the ultrastructural level using transmission electron microscopy (TEM) of the synaptic regions of SCM and soleus muscle ( Fig 3a–f ). Interestingly, the NMJs in the SCM of MCK mice not only exhibited more folds per individual synapse ( Fig. 3a ) but also a significant increase in the average length of these synaptic folds ( Fig. 3b ), as illustrated by a representative TEM picture shown in Fig. 3c . To confirm the increase in fold density in the NMJ from MCK NMJs, we measured the expression of the Na V 1.4 channel concentrated in the depths of the folds using western blot ( Fig. 3d , see Supplementary Fig. 1 for representative full-sized western blots). The expression of Na V 1.4 was correlated with the fold quantification, being higher in the muscle of transgenic animals. In contrast, the number and average length of the synaptic folds in soleus muscle of the MCK mice were not different from those of the WT controls ( Fig. 3e,f , respectively) correlating with the difference in PGC-1α expression in SCM but not the soleus of MCK compared with WT mice. Figure 3: Synaptic fold characterization on the TEM images from WT and transgenic mice NMJs. ( a ) The average number of folds attached to synapses was determined for WT and MCK mice in SCM muscle. ( b ) Synaptic fold lengths from SCM muscles were scaled and measured with Image J and averaged. Each bar represents mean±s.e.m. ( n =4, t- test two-tailed). ( c ) Representative TEM image of the NMJ area of SCM muscle from WT or MCK animals. ( d ) Western blot detection of the Na v 1.4 expression in SCM muscles from WT and MCK animals. The relative band intensity was analysed using the Image J. The WT/tubulin ratio was set as 100%. ( e ) The average number of folds attached to synapses was determined for WT and MCK mice in soleus muscle. ( f ) Synaptic fold lengths from soleus muscles were scaled and measured with Image J and averaged. Each bar represents mean±s.e.m. ( n =4, t- test two-tailed). SF: Synaptic folds, m: mitochondria. Full size image Muscle PGC-1α promotes slow-type NMJ function The morphological and ultrastructural analysis of the NMJ in MCK versus WT mice not only suggests stabilization but also a shift towards slow-type NMJs in the MCK mice—for example, indicated by the smaller end plate size in these animals. As a next step, we therefore wanted to test whether the morphological changes induced by overexpressed PGC-1α in the skeletal muscle were sufficient to trigger functional adaptations of motor neuron–muscle fibre interaction. First, compound muscle action potentials in response to repetitive nerve stimulation were assessed by electromyography. Specifically, the train of compound action potentials following direct stimulation of the sciatic nerve with a frequency of 50 Hz was recorded in the gastrocnemius of WT and MCK animals ( Fig. 4a,b , respectively). Interestingly, while the amplitude of the first response was similar in the MCK and WT animals, the amplitude and area under the curve of the successive responses showed a significant decrement in the WT animals that was much lower in the MCK mice ( Fig. 4c ). 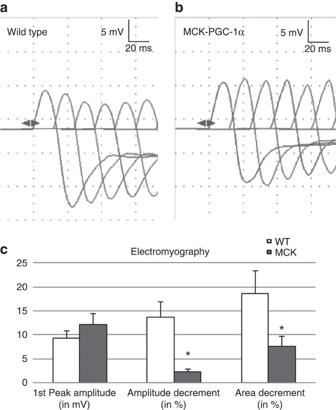Figure 4: Electromyographic properties of the gastrocnemius muscles in WT and MCK mice after repetitive nerve stimulation of the sciatic nerve. (a,b) Representative electromyography traces of WT (a) and MCK mice (B). (c) Average of the first peak amplitude in mV and the decrement (amplitude and area) calculated between the first and the fourth peaks of the train of action potentials recorded in WT (white bars) and MCK animals (grey bars). Each bar represents mean±s.e.m. *P<0.05 (n=7,t-test two-tailed). Figure 4: Electromyographic properties of the gastrocnemius muscles in WT and MCK mice after repetitive nerve stimulation of the sciatic nerve. ( a , b ) Representative electromyography traces of WT ( a ) and MCK mice (B). ( c ) Average of the first peak amplitude in mV and the decrement (amplitude and area) calculated between the first and the fourth peaks of the train of action potentials recorded in WT (white bars) and MCK animals (grey bars). Each bar represents mean±s.e.m. * P <0.05 ( n =7, t- test two-tailed). Full size image To refine the functional studies, we subsequently investigated neurotransmission at the NMJ of the glycolytic LAL, which exhibits similar morphological NMJ plasticity in MCK mice to the leg glycolytic muscles and the oxidative TVA muscle with unchanged morphological properties between the two genotypes ( Supplementary Fig. 2 ). First, we measured muscle resting membrane potential and found no significant differences between MCK and WT mice in either muscle ( Supplementary Table 1 ). Then, when studying the spontaneous miniature end-plate potentials (mEPP) in LAL, a significantly slower mEPP rise time in MCK mice (0.78±a s.d. of 0.03 s) in comparison with WT (0.68±a s.d. of 0.02 s) was observed ( P =0.03, t- test), while no significant differences in mEPP amplitude, frequency or signal decay constant were found ( Fig. 5a ). Similarly, the rising time of evoked endplate potentials (EPPs) in the LAL of MCK mice was significantly slower (0.75±a s.d. of 0.02 s) than in WT (0.66±a s.d. of 0.02 s; P =0.0085), while the amplitude and decay time constant of the EPPs remained unchanged in MCK mice ( Fig. 5b ). As EPPs are slower in slow muscles than in fast muscles [31] , we next measured the properties of mEPPs and EPPs in the oxidative TVA muscle ( Supplementary Fig. 3 ). As expected, the mean rising times of mEPPs and EPPs in WT TVA were slower than in WT LAL muscles ( Tables 1 and 2 ) but not significantly different to those values measured in MCK LAL muscles. On the other hand, no difference in the rising times of spontaneous and evoked potentials was found between WT and MCK mice in the TVA ( Tables 1 and 2 ). 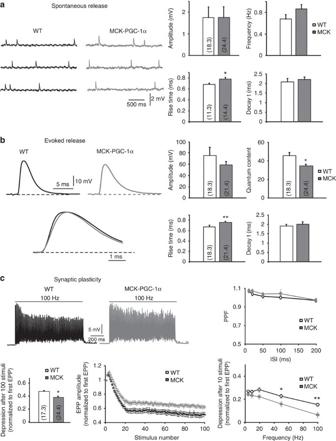Figure 5: Electrophysiological properties of LAL muscles from WT or transgenic mice (a) The spontaneous neurotransmitter release of LAL muscle resembled the representative traces of mEPP in WT (black) and MCK-PGC-1α (gray) NMJs. Amplitude, frequency of mEPP and their rise and decay times were determined. (b) Evoked neurotransmitter release resembled the representative traces of EPP in WT (black) and MCK-PGC-1α (grey) NMJs. Amplitude, quantum content of EPP and their rise and decay times were determined. (c) The synaptic plasticity shows a representative trace of steady-state depression in WT (black) and MCK-PGC-1α (grey) mice. The pair-pulse-facilitation (PPF) at inter-stimulus-intervals (ISI) ranging from 10 to 200 ms and the steady-state depression were measured at the end of the train and normalized to the amplitude of the first EPP. The normalized depression after 10 repetitive stimuli was measured between 0 and 100 Hz. The results are represented as mean±s.e.m. The numbers in the bars aren,N: number of fibres, number of mice. Figure 5: Electrophysiological properties of LAL muscles from WT or transgenic mice ( a ) The spontaneous neurotransmitter release of LAL muscle resembled the representative traces of mEPP in WT (black) and MCK-PGC-1α (gray) NMJs. Amplitude, frequency of mEPP and their rise and decay times were determined. ( b ) Evoked neurotransmitter release resembled the representative traces of EPP in WT (black) and MCK-PGC-1α (grey) NMJs. Amplitude, quantum content of EPP and their rise and decay times were determined. ( c ) The synaptic plasticity shows a representative trace of steady-state depression in WT (black) and MCK-PGC-1α (grey) mice. The pair-pulse-facilitation (PPF) at inter-stimulus-intervals (ISI) ranging from 10 to 200 ms and the steady-state depression were measured at the end of the train and normalized to the amplitude of the first EPP. The normalized depression after 10 repetitive stimuli was measured between 0 and 100 Hz. The results are represented as mean±s.e.m. The numbers in the bars are n , N : number of fibres, number of mice. Full size image Table 1 Spontaneous neurotransmitter release in NMJs of LAL and TVA muscles. Full size table Table 2 Evoked neurotransmitter release in NMJs of LAL and TVA muscles. Full size table Short-term synaptic plasticity at the NMJ of the LAL muscle was tested by repetitive trains of stimuli of 1 s at 100 Hz ( Fig. 5c ). No differences in paired-pulse ratio at interstimulus intervals ranging from 10 to 200 ms were observed between the genotypes ( Fig. 5c ), suggesting no differences in synaptic release probabilities. In contrast, steady-state depression at the end of the 1 s, 100-Hz train of stimuli were significantly lower in the MCK (39±a s.d. of 2%) compared with WT (48±a s.d. of 3%) mice ( P =0.03, t- test; Fig. 5c ). The ability of the MCK motor neuron terminals to sustain neurotransmitter release more efficiently than their WT counterparts became evident even after a few stimuli. For example, smaller depression after 10 repetitive stimuli was observed in the MCK mice, as a trend at 20 Hz ( P =0.054, t- test), and with statistical significance at 50 Hz ( P =0.014, t- test) and 100 Hz ( P =0.004, t- test; Fig. 5c ). In motor nerve fibres that innervate slow (type I) muscle fibres neurotransmitter release is better sustained than in nerve terminals that innervate fast muscle fibres. This has been attributed to a larger synaptic vesicle pool size and lower quantal content (the number of quanta of neurotransmitter released per action potential) in slow motor neurons [23] . Therefore, we next compared the quantum content in the LAL of MCK and WT animals ( Fig. 5b ) and found that it was significantly smaller in MCK (34.7±a s.d. of 1.8) than in WT (45.8±a s.d. of 3.6) terminals ( P =0.01, t- test). Therefore, the reduction in the number of fused vesicles per action potential, probably, contributed to less depression in MCK LAL terminals. This compensation was further confirmed when the cumulated number of fused synaptic vesicles during 100-Hz stimulation was calculated in both genotypes and not statistical differences were obtained ( Supplementary Table 2 ). Finally, we also estimated size of the readily releasable pool of synaptic vesicles [32] in the nerve terminals of the LAL and found no differences between MCK and WT mice ( Supplementary Table 3 ), suggesting that if the overexpression of PGC-1α induces an increase of synaptic vesicles that should be at the level of the reserve pool and not at the readily releasable pool. In the oxidative TVA, a significant increase in the amplitude of the spontaneous mEPPs as well as an increase in the decay time constant of the evoked EPPs was found in MCK mice ( Supplementary Fig. 3 ). Finally, short-term depression after 10 repetitive stimuli at 50 Hz was reduced in the TVA of MCK animals compared with WT animals, while the rest of the electrophysiological parameters did not differ significantly between the genotypes in this muscle ( Supplementary Fig. 3 ). Pre-synaptic remodelling of the NMJ by PGC-1α The functional data obtained by the single motor neuron–muscle fibre-based electrophysiology strongly implies that the nerve endplates in the MCK animals with muscle-specific overexpression of PGC-1α not only undergo a post-synaptic but also a pre-synaptic remodelling. To substantiate this hypothesis, we studied the pre-synapse in more detail. Quantification of the nerve terminal branches within the region of the NMJ revealed a significantly higher number in nerve branches as well as an increased total length and branching complexity in the SCM of MCK animals compared with WT mice ( Fig. 6a ). These findings indicate a change in the pre-to-post-synaptic coupling in the PGC-1α muscle-specific transgenics. In fact, increased length of branching is usually accompanied by an increase in the number of ACh-containing vesicles in the pre-synaptic part in order to store more neurotransmitter. First, we quantified the number of synaptic vesicles using TEM ( Fig. 6b ). We observed a significantly higher number of synaptic vesicles in nerve terminals of the glycolytic SCM muscle of MCK mice compared with WT animals but no significant differences in terminals from the oxidative soleus muscle ( Fig. 6c ). Interestingly, the protein expression of synaptophysin (Syp), a pre-synaptic regulator of vesicle fusion, was likewise differentially expressed in the TA and SCM of MCK animals compared with WT mice ( Fig. 6d ). It was previously shown that the overexpression of PGC-1α in the muscle increased the frequency of motor neuron expressing the synaptic vesicle protein SV2A [34] . By isolating the synaptic area in the SCM muscle, we could confirm an increase in the expression of this protein in the MCK samples compared with their WT counterparts ( Fig. 6e ). 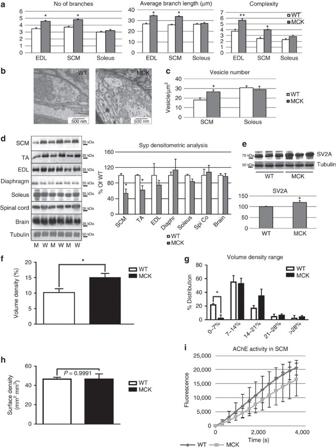Figure 6: Pre-synaptic remodelling of the NMJ by PGC-1α. (a) The number of branches per AChR cluster and the average length of the branches were determined on confocal images stack using Image J in arbitrary units on WT (white bars) and MCK (grey bars) mice. The complexity is defined as the branch number × the total branch length divided by 100. Each bar represents mean±s.e.m. from at least 100 NMJ from three mice *P<0.05 **P<0.01 (N=3,n>100,t-test two-tailed). (b) Representative TEM picture illustrating the synaptic vesicle number in the SCM muscle from WT and MCK mice. (c) Quantification of synaptic vesicle number per μm2determined by Image J on WT (white bars) and MCK (grey bars) mice. Each bar represents mean±s.e.m. from at least 10 NMJ from three mice *P<0.05 (N=3,n>10,t-test two-tailed. (d) Western blot detection of synaptophysin on protein extracts from different tissues of WT (W, white bars) and MCK (M, grey bars) animals. The relative band intensity was analyzed by Image J. The WT/tubulin ratio was set as 100%. *P<0.05 (N=3). (e) Western blot detection of the synaptic vesicle 2A on SCM protein extract in WT and MCK mice. (f,g) Volume density of mitochondria within the NMJ was calculated according to Weibel33using a D64 grid (q2=16,PT=64,P′T=1024) at × 8,500 magnification. Individual NMJ data (N=9–16 per mouse) were averaged per mouse and subsequently between mice at the same genotype (WT=4, MCK=3). Unpairedt-test. (h) The surface density of mitochondria (right) was calculated according to Weibel using a customized D576 Grid (q2=16,PT=576,P’T=9216) at × 8500 magnification. Individual NMJ data (N=9–16 per mouse) were averaged per mouse and subsequently between mice at the same genotype (WT=4, MCK=3). Unpairedt-test. (i) For SCM muscle, a kinetic of AChE activity was measured indirectly by detecting the fluorescence emitted at 590 nm for 3,600 s. Each point represents mean±s.e.m. (N=3). Figure 6: Pre-synaptic remodelling of the NMJ by PGC-1α. ( a ) The number of branches per AChR cluster and the average length of the branches were determined on confocal images stack using Image J in arbitrary units on WT (white bars) and MCK (grey bars) mice. The complexity is defined as the branch number × the total branch length divided by 100. Each bar represents mean±s.e.m. from at least 100 NMJ from three mice * P <0.05 ** P <0.01 ( N =3, n >100, t- test two-tailed). ( b ) Representative TEM picture illustrating the synaptic vesicle number in the SCM muscle from WT and MCK mice. ( c ) Quantification of synaptic vesicle number per μm 2 determined by Image J on WT (white bars) and MCK (grey bars) mice. Each bar represents mean±s.e.m. from at least 10 NMJ from three mice * P <0.05 ( N =3, n >10, t- test two-tailed. ( d ) Western blot detection of synaptophysin on protein extracts from different tissues of WT (W, white bars) and MCK (M, grey bars) animals. The relative band intensity was analyzed by Image J. The WT/tubulin ratio was set as 100%. * P <0.05 ( N =3). ( e ) Western blot detection of the synaptic vesicle 2A on SCM protein extract in WT and MCK mice. ( f , g ) Volume density of mitochondria within the NMJ was calculated according to Weibel [33] using a D64 grid ( q 2 =16, P T =64, P ′ T =1024) at × 8,500 magnification. Individual NMJ data ( N =9–16 per mouse) were averaged per mouse and subsequently between mice at the same genotype (WT=4, MCK=3). Unpaired t- test. ( h ) The surface density of mitochondria ( right ) was calculated according to Weibel using a customized D576 Grid ( q 2 =16, P T =576, P ’ T =9216) at × 8500 magnification. Individual NMJ data ( N =9–16 per mouse) were averaged per mouse and subsequently between mice at the same genotype (WT=4, MCK=3). Unpaired t- test. ( i ) For SCM muscle, a kinetic of AChE activity was measured indirectly by detecting the fluorescence emitted at 590 nm for 3,600 s. Each point represents mean±s.e.m. ( N =3). Full size image Importantly, both acetylcholine biosynthesis and synaptic vesicle assembly are energy-consuming processes. To assess whether the structural and functional changes of the pre-synapse are accompanied by a corresponding adaptation of the metabolic properties, mitochondrial size and morphology were quantified with TEM. Intriguingly, a significant increase in the mitochondria volume density was observed in the transgenic animals ( Fig. 6f ). This was accompanied by a prominent reduction in the number of mitochondria of the smallest volume density range, which was compensated by an increase in the proportion of mitochondria with a high volume density ( Fig. 6g ). In contrast, no statistically significant difference in average surface (cristae) density was found ( Fig. 6h ). Strikingly, even in the oxidative soleus muscle, a significant increase in pre-synaptic mitochondrial volume density was observed, while mitochondrial surface density was unchanged in the active zone of the motor neuron innervating Soleus ( Supplementary Fig. 4 ). After pre-synaptic acetylcholine release, relative acetylcholine esterase activity in the neuromuscular cleft determines the rate of neurotransmitter breakdown and hence removal from the cleft. In contrast to the clear pre- and post-synaptic differences, acetylcholine esterase activity in the synaptic cleft is statistically indistinguishable between the two genotypes in any of the muscles studied ( Fig. 6i and Supplementary Fig. 5 ). In the mature skeletal muscle tissue, activity-driven plasticity is the most important cause for NMJ remodelling [12] . Nevertheless, despite the well-documented modulation of NMJ structure and morphology in response to altered neuromuscular activity, very little is known about the molecular processes that control this type of NMJ plasticity. Historically, altered firing patterns of the motor neuron have been implicated as an exclusive source of the remodelling of the neuromuscular interface and the ensuing adaptations in the muscle fibre [35] —that is, a switch towards oxidative and glycolytic muscle fibres caused by altered intramyocellular calcium transients in endurance and resistance training, respectively [15] . In contrast to the developmental aspects of NMJ installation, the contribution of skeletal muscle fibres to these adaptive processes has been only rudimentarily studied. In recent years however, our understanding of the molecular mechanisms that underlie skeletal muscle cell plasticity has been tremendously expanded. For example, skeletal muscle is now widely recognized as an endocrine tissue that releases auto-, para- and endocrine hormones, so-called myokines [36] . Furthermore, we could show that intramyocellular calcium handling is not only controlled by motor neuron input but also cell autonomously modulated by PGC-1α [30] . In the present study, we now provide strong evidence of a significant contribution of skeletal muscle to pre- and postsynaptic remodelling of the NMJ through elevated activity of the coactivator PGC-1α. In mice with skeletal muscle-specific overexpression of PGC-1α, the NMJ is altered morphologically, structurally and functionally despite unchanged locomotion and hence motor neuron-mediated activation of muscle fibres. Moreover, these mice exhibit a similar muscle fibre size distribution as control animals [37] : a change in fibre size thus is not the underlying cause of altered NMJ properties. Importantly, the extent of the plastic changes correlates with the relative overexpression of PGC-1α in muscles with different fibre-type characteristics. For example, major rearrangements of the NMJs are found in the glycolytic SCM with high transgenic overexpression of PGC-1α compared with the minor alterations in the oxidative soleus where transgenic elevation of PGC-1α is minimal. Morphology and function of the NMJs in the MCK mice resemble those of slow-type NMJs innervating oxidative muscle beds—for example, as indicated by the smaller endplate size [38] . Functionally, this switch towards slow-type NMJs allows a more sustained firing pattern that is typical for the high endurance contractions in slow muscles, at least in part by a higher number of synaptic vesicles and increased mitochondrial volume density in the active zone combined with a smaller quantum content. This modulation in synaptic vesicle handling in the active zone of the motor neuron is further underlined by the distinct expression of proteins involved in synaptic vesicle function such as synaptophysin and the slow-type NMJ-enriched synaptic vesicle protein 2A (SV2A), which has previously been reported to be increased in NMJs of MCK animals [34] . Similarly, the changes in kinetics of the mEPPs and EPPs, in particular the increase in rise time, are typical for slow-type NMJs [31] , [39] . Finally, our data also reveal the increase in pre-synaptic nerve terminal branching that is linked to activity-driven adaptations of the NMJ [12] , [17] . Importantly, the reduction in quantum content is not indicative of failure in neurotransmission, given the high safety factor in the NMJ, the unchanged high amplitude of the post-synaptic end-plate potential, the reduced depression in the amplitude of the responses following repetitive nerve stimulation in the EMG and in the intracellular recordings and finally illustrate the fatigue resistance in PGC-1α-overexpressing muscles in and ex vivo . Thus, muscle PGC-1α induces many post- and, importantly, pre-synaptic changes that have been linked to activity-driven NMJ plasticity in the adult muscle. The large amplitude of the EPP that we observe may be related with the mouse background. In our experience, and in that of others, EPP amplitude in mice with a C57BL/6 background have larger EPP than FVB mice [40] . This large amplitude was also confirmed in a number of fibres in which two-electrode voltage clamp recordings were obtained. Typical peak currents in WT mice were 70–80 nA, while the mean input resistance was 0.84 MΩ. This results in EPP amplitudes of 58–68 mV. Intriguingly, PGC-1α-mediated modulation of NMJ morphology also closely resembles the beneficial effects of caloric restriction and exercise on age-related deterioration of the neuromuscular interface [18] . Thus, we observed an improvement in morphological NMJ integrity both in post-synaptic features such as AChR density and pretzel fragmentation, as well as pre-synaptically in terms of innervation and sprouting. On the ultrastructural level, the increase in synaptic fold number and length in the MCK animals indicates a structural stabilization as well as an enhancement of the synaptic transmission triggered by overexpressed muscle PGC-1α [41] . Interestingly, exercise affects only the NMJs of a subgroup of aged muscles whereas the effect of caloric restriction is more ubiquitous [18] . Similarly, muscle-specific overexpression of PGC-1α had distinctive outcomes on NMJ morphology and function in different muscles. In our experimental context of sedentary mice, these differences could be caused by the relative usage of the muscles that were characterized in the animals. It thus might be interesting in future studies whether bona fide exercise of the MCK mice extends the remodelling of the NMJs beyond those that were observed in the sedentary animals. A corresponding amplification of muscle-specific transgenic expression of PGC-1α by treadmill running has previously been reported in regard to diet-induced peripheral insulin resistance [42] . Our finding that muscle PGC-1α not only remodels the post-synapse, but also triggers a significant pre-synaptic adaptation of the NMJ obviously suggest the production of a PGC-1α-dependent neurotrophic factor that mediates a local, retrograde signal from muscle to the motor neuron. While a number of retrograde signals have been identified in the formation of NMJs during development, very little about the role of skeletal muscle and hence about putative retrograde signaling mediators is known in physiological NMJ plasticity in the adult muscle. We have tested some candidate retrograde signaling molecules that have been described in the context of developmental NMJ differentiation [2] , including several extracellular matrix components, but did not observe any differences in gene expression between MCK and WT mice ( Supplementary Fig. 6 ). Therefore, it is conceivable that different factors convey a retrograde signal in the mature compared with the developing NMJ. However, while we would expect a transcriptional response due to overexpression of the transcriptional coactivator PGC-1α, our findings obviously do not exclude post-transcriptional mechanisms to contribute to retrograde signalling in our experimental context. Similarly, the increase in PGC-1α-mediated AChR expression and clustering, MuSK or some other post-synaptic protein might contribute to the retrograde signaling. Nevertheless, it is also possible that so far uncharacterized neurotrophic factors could be involved in physiological NMJ plasticity and future studies will aim at identifying those. In summary, we now for the first time provide strong evidence for a significant contribution of skeletal muscle to physiological NMJ plasticity in adult muscle, both on the post- as well as on the pre-synaptic side. In particular, it is conceivable that PGC-1α, a regulatory nexus in metabolic and myofibrillar endurance exercise adaptation in muscle, also controls activity-dependent remodeling of the NMJ and contributes to the attenuation of the age-related deterioration of neuromuscular morphology and function by exercise. PGC-1α has previously been described to ameliorate muscle atrophy and fibre damage in different pathological contexts, including Duchenne muscular dystrophy [20] . In Duchenne muscular dystrophy, NMJ dysfunction is thought to contribute to the disease pathology. While the exact mechanism by which skeletal muscle-specific overexpression of PGC-1α improves muscle fibre integrity and function in mdx animals, the mouse model for Duchenne muscular dystrophy, PGC-1α-mediated stabilization of the NMJ could certainly be a part of this therapeutic effect. Similarly, the prevention of sarcopenia in muscle-specific PGC-1α transgenic mice could be due to the functional improvement in the NMJ as has been shown in old animals [27] . In contrast, skeletal-muscle-specific overexpression of PGC-1α ameliorated the muscle pathology of an amyotrophic lateral sclerosis mouse model, but was insufficient to extend survival [29] . These findings indicate that the effect of muscle PGC-1α on NMJ stability might be insufficient in very severe motor neuron diseases, but could be therapeutically beneficial in pathologies with a milder motor neuron phenotype or with secondary deterioration of the NMJ. Therefore, identification of pharmacological agents that activate PGC-1α in human muscle or that target the muscle-derived factors, which mediate the retrograde signaling in this context, is of high clinical importance. Thus, similar to our current understanding of the potential deployment of “exercise mimetics” in the treatment of metabolic diseases, such compounds might also be excellent adjuvant interventions to facilitate and bona fide exercise in patients with impaired exercise tolerance. Animals All experiments were performed on male, 6- to 8-week-old wild-type (WT) and transgenic mice (all mice obtained from in-house breeding) where the PGC-1α expression is driven by a muscle creative kinase (MCK) promoter (designated MCK mice, as opposed to the WT littermates) [22] . The animals were kept in a room with a 12/12 light/dark cycle, were fed a standard laboratory chow diet and had ad libitum access to water. All animal experiments were approved by the institutional as well as Swiss cantonal veterinary authorities according to the guidelines of the European Council Directive for the Care of Laboratory Animals. Tissue preparation Isolated muscles were directly frozen in liquid nitrogen. Total RNA was extracted using TriReagent according to the the manufacturer’s protocol and was treated with RNase-free DNase (Invitrogen). The concentration was adjusted and 1 μg of RNA was reverse-transcribed into cDNA using Superscript RT (Invitrogen) with random hexamer primers (Roche). Real-time PCR was performed with the Power Sybr Green Master Mix (Applied Biosystems) using the StepOne Plus Lightcycler (Applied Biosystems). The relative expression level for each gene of interest was estimated according to the ΔΔ C t method, using the WT samples as reference and the expression of the TATA-binding protein as a calibrator. Real-time PCR primers are shown in Supplementary Table 4 . For protein extraction, the frozen muscles or tissues were digested with lysis buffer (Tris HCl 20 mM, NaCl 138 mM, KCl 2.7 mM, Glycerol 5% v/v, NP40 1% v/v) supplemented with a cocktail of protease inhibitors (Roche) and the protein concentration was quantified with the BCA protein assay kit (Pierce, Thermofisher). Proteins were resolved by SDS-PAGE, transferred to a polyvinylidene difluoride membrane and incubated with an anti-synaptophysin antibody (Abcam, Ref. ab53166, 45 kD), anti-SCN4A antibody (Novus Biological, Ref NBP1–19008, 208 kDa) and SV2A antibody (Novus Biological, Ref NBP1-46367, 88 kD). Tubulin expression (Upstate Cell Signaling, Ref 05–829, 55 kDa) was used as loading control. The relative intensity of the bands of interest was analysed using Image J and was expressed relative to the tubulin band intensity. The WT/tubulin level was set as 100%. To be able to measure the expression of pre-synaptic markers from the muscle samples, the synaptic part was stained with Alexa Fluor 488-coupled α-bungarotoxin and micro-dissected under a binocular microscope. The isolated synaptic part was then processed as other samples for protein or RNA extraction. For immunofluorescence, soleus, EDL, diaphragm and SCM were isolated. The collected muscles were fixed for 10 min at −20 °C in methanol, washed in phosphate-buffered saline and incubated for 2 h at room temperature in a blocking solution (phosphate-buffered saline supplemented with 1% bovine serum albumin, 5% Horse serum, 1% Triton-X100, 0.1% NaN3). The whole muscles were then incubated overnight at 4 °C with a mixture of primary antibody and Alexa Fluor 488-coupled α-bungarotoxin (Molecular Probe, Ref B13422) diluted 1/10,000 in blocking solution. The polyclonal antibody against the neurofilament (Chemicon-millipore, Ref AB1987) was used at a 1/1,000 dilution and the polyclonal anti-synaptophysin (Dakocytomation Ref M7315) at 1/200. After 4 h of incubation with the adequate secondary antibodies, the muscles were whole-mounted on slides with a fluorescent mounting medium (Dako). The samples were observed under a confocal microscope (DMI6000, Leica) and maximum intensity projections of stacks were used to study the NMJ structure. The same settings were kept for all the samples (thickness of the scanned area, number of layers, gain and offset). The NMJ architecture characterization was based on the definitions given by Sanes and Lichtman [18] . More than 100 NMJs ( n ) from at least three animals ( N ) were counted. Pre-synaptic variables of NMJ included the number of branches identified at the nerve terminal, the total length of those branches, the average length per branch and the branching complexity obtained by multiplying the number of branches by the total length of those branches, and dividing that figure by 100 as described previously [43] . For electrophysiology recordings, the LAL and TVA muscles were dissected with their nerve branches intact and pinned to the bottom of a 2-ml chamber, over a bed of cured silicon rubber (Sylgard, Dow Corning. Preparations were continuously perfused with a solution of 125 mM NaCl, 5 mM KCl, 2 mM CaCl 2 , 1 mM MgCl 2 , 25 mM NaHCO 3 and 15 mM glucose under a continuous flow of a 5% CO 2 /95% O 2 gas mixture. Synaptic fold quantification Synaptic fold lengths were determined for individual NMJs using the Image J software and TEM images at × 8,500 magnification. Lengths were measured cursively from the edge of the synapse to the end of each fold using a Wacom CTH-470 pen tablet. Synaptic fold lengths and synaptic fold number per NMJ ( N =9–16 per mouse) were averaged per mouse and subsequently between mice at the same genotype (WT=4, MCK=4 in SCM muscle). Volume and surface density of pre-synapse Volume and surface density of mitochondria within the NMJ were calculated according to methods previously described by Weibel [33] and digitally adapted to Adobe Photoshop. Mitochondria and cristae structures within the NMJ were identified and outlined manually using a Wacom CTH-470 pen tablet. Volume density was determined in a test point system utilizing a D64 grid ( q 2 =16, P T =64, P ’ T =1024) using TEM images of × 8,500 magnification. Volume density ( V V ) is defined in the equation 1 as the ratio of test points residing within mitochondria ( P M ) and the total amount of test points within the NMJ ( P NMJ ). Cristae density of mitochondria was measured at equal magnification in a test point system using a D576 grid ( q 2 =16, P T =576, P ’ T =9216). Cristae density of individual mitochondria ( S V(cr,mt) ) is defined in equation 2 as the total amount of intersections between inner mitochondrial membrane and test lines ( I cr ) divided by the product of the amount of points within the mitochondria ( P mt ) and the actual length of fine test lines in μm (d). Cristae density was determined in one mitochondrion randomly selected in each NMJ for a total of 9–16 NMJ per mouse. NMJ data for cristae and volume density were averaged per mouse and subsequently between mice at the same genotype (WT=4, MCK=3 in SCM muscle). AChE enzymatic activity measurement The AChE activity was measured using the Amplex Red Acetylcholine/Acetylcholinesterase Assay Kit (Molecular Probes). Each reaction contained 200 μM Amplex Red Reagent containing 1 U ml −1 HRP, 0.1 U ml −1 choline oxidase and 100 μM acetylcholine. The choline generated from AChE activity is oxidized by choline oxidase to betaine and H 2 O 2 that reacts with the Amplex Red reagent to generate a fluorescent product detected at 590 nm ( N =3 for each experimental group). Electromyography Mice were anesthetized using sevofluorane. The electromyographic properties of the gastrocnemius were recorded using a Keypoint EMG machine (Meridian, Neurolite AG, Switzerland). Briefly, the sciatic nerve was directly repetitively stimulated by a train of 15 stimulations (0.04 ms of duration, 10 mA of amplitude) in a supramaximal conditions at 50 Hz with two monopolar needle electrodes and the action potentials in the gastrocnemius muscle response were recorded using a needle electrode placed directly in the muscle belly. The decrement percentage in terms of amplitude and area was averaged for WT and MCK mice ( N =4 for each experimental group). Electrophysiology The electrical stimulation and intracellular recording were performed as previously described [44] . Briefly, the nerve was stimulated by means of a suction electrode. The stimulation consisted of square-wave pulses at variable frequencies. A glass microelectrode filled with 3 M KCl was connected to an intracellular recording amplifier (Neuro Data IR283, Cygnus technology) and used to impale single muscle fibres near the motor nerve endings. EPP and mEPPs were recorded from different NMJs within the muscle as described previously. Muscle contraction was prevented by including in the bath 3–4 μM μ-conotoxin GIIIB (Alomone Laboratories), a specific blocker of muscular voltage-gated sodium channels. The data were analysed as previously described [44] . EPP amplitudes were normalized to −70 mV and corrected for nonlinear summation. Transmission electronic microscopy The samples were prepared and processed by the Center for Microscopy of the Basel University (ZMB, Basel, Switzerland). The muscles were fixed in a 3% paraformaldehyde, 0.5% glutaraldehyde-buffered solution for 1 h and subsequently incubated in a 1% osmium tetroxide-buffered solution. The slides were dehydrated in a graded EtOH series (50–100%), infiltrated in 100% acetone, embedded in Epon and serially thin-sectioned before staining with uranyl acetate and lead acetate. The samples were analysed on a transmission electronic microscopy Moragni 268D (Philips) at 80 kV. Statistical analysis The results are represented as mean±s.e.m., unless otherwise stated. The MCK and WT samples were compared using the Student’s t- test (two-tailed) and a P -value <0.05 was considered statistically significant. N =number of mice, n =number of pretzels or number of fibres. How to cite this article: Arnold, A.-S. et al. Morphological and functional remodeling of the neuromuscular junction by skeletal muscle PGC-1α. Nat. Commun. 5:3569 doi: 10.1038/ncomms4569 (2014).